Discreteness-induced concentration inversion in mesoscopic chemical systems Molecular discreteness is apparent in small-volume chemical systems, such as biological cells, leading to stochastic kinetics. Here we present a theoretical framework to understand the effects of discreteness on the steady state of a monostable chemical reaction network. We consider independent realizations of the same chemical system in compartments of different volumes. Rate equations ignore molecular discreteness and predict the same average steady-state concentrations in all compartments. However, our theory predicts that the average steady state of the system varies with volume: if a species is more abundant than another for large volumes, then the reverse occurs for volumes below a critical value, leading to a concentration inversion effect. The addition of extrinsic noise increases the size of the critical volume. We theoretically predict the critical volumes and verify, by exact stochastic simulations, that rate equations are qualitatively incorrect in sub-critical volumes. Mesoscopic chemical reaction systems are typically realized in compartments with length scales ranging from few tens of nanometers to millimeters. The same concentration realized in compartments of decreasing size implies a decreasing total number of molecules. This leads to an increase in apparent molecular discreteness and an increase in the size of the concentration fluctuations about the mean [1] . These intrinsic fluctuations stem from the discrete change in the number of molecules when a reaction occurs, and their random character is principally imparted by the contact of the system with a heat bath [2] . Chemical reaction dynamics in small-scale compartments is hence considerably influenced by intrinsic (or internal) noise. Biological cells are natural and ubiquitous examples of highly confined chemically reactive systems. Biochemical reactions proceed in sub-micron compartments where the total number of molecules is in the range of one to several thousand [3] , [4] , and intrinsic noise is hence expected to have an important functional role in biochemical circuits [5] . Biological systems are also subjected to extrinsic noise originating outside the immediate system of interest. For example, the rate of chemical reactions inside a compartment may depend on the abundance of an upstream species that is translocated from another compartment [6] , [5] . The relevance of intrinsic noise, however, is not limited to biological systems. Molecular capsules [7] , carbon nanotubes [8] and crystalline zeolites [9] are other examples of nanospaces confining chemical reactions. It has been shown that accounting for intrinsic noise leads to a considerable modification of the temperature dependence of the equilibrium constants of reactions in such confined spaces [10] . There is an extensive literature on modelling the effects of intrinsic noise in chemical kinetics. Intrinsic noise is taken into account by chemical master equations (CMEs), which are exact mesoscopic descriptions of well-stirred and thermally equilibrated gas-phase chemical systems [11] and chemical reactions occurring in well-stirred dilute solutions [12] . Unfortunately, CMEs are generally analytically intractable, and many studies have therefore resorted to the linear-noise approximation (LNA) of the CME (see, for example, refs 13 , 14 , 15 , 16 , 17 , 18 , 19 ). The LNA prediction of mean concentrations is the same as that from rate equations (REs) [20] , [21] , but it is well known that, for systems involving at least one bimolecular reaction, the mean concentrations approach those from the REs only in the macroscopic limit of large molecule numbers [1] , [22] , [23] . Hence, the LNA cannot capture effects in the mean that are due to molecular discreteness. Recently, it has also been shown that the relaxation kinetics around steady states of nonlinear reactions is altered by molecular discreteness [24] , [25] . It is thus likely that the functionality and operation of chemical circuits involving low copy numbers of some species may considerably differ from standard predictions based on the LNA or REs. In addition, a detailed understanding of how extrinsic noise influences a circuit's low-copy-number properties is desirable because experimental studies suggest that extrinsic noise is frequently comparable to, or larger than, intrinsic noise [26] . Here we investigate the dependence of the non-equilibrium steady-state properties of a monostable nonlinear chemical circuit on the discreteness of the interacting molecules. We consider independent realizations of the same chemical reaction system in compartments of different volumes. Given some fixed-rate constants, the LNA and REs predict the same steady-state concentrations for all realizations. In contrast, we show that accounting for molecular discreteness leads to volume-dependent steady-state mean concentrations, and that the RE and LNA predictions are qualitatively correct only for systems above a critical volume. This describes a new phenomenon: discreteness-induced concentration inversion. For systems in sub-critical volumes, the REs and LNA predict that the steady-state mean concentration of a species A is, say, larger than that of another species B, whereas accounting for discreteness leads to the reverse prediction. We present a theory to explain this novel discreteness-induced inversion effect and to predict the values of the critical volumes. We illustrate and validate the theory by comparing its predictions to exact stochastic simulations of the CME for the generic model system of trimerization ( Fig. 1 ). Furthermore, we show that the critical volume increases in the presence of extrinsic noise due to bursty input of a reactant into the compartment. 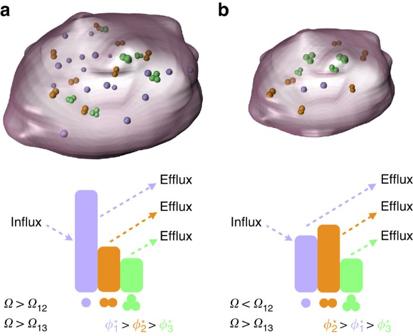Figure 1: Discreteness-induced inversion effect. The species are monomers (species 1, purple), dimers (species 2, orange), and trimers (species 3, green). They are involved in an open trimerization reaction confined to a compartment of volumeΩ. Monomers enter the compartment, bind to other monomers to form dimers, and to dimers to form trimers. All molecules leave the compartment at a constant rate. The spheres represent the molecules, whereas the semi-transparent pink surface represents the arbitrarily shaped compartment to which the molecules are confined. The bar graphs reflect the steady-state mean concentrations (denotedfor speciesi). When the volume decreases below a critical valueΩ12, the ratio of the steady-state mean concentrations of monomers (species 1) and dimers (species 2) changes from greater than one to less than one. This inversion effect is induced by an increase in the apparent discreteness of the system as the volume is decreased from (a) to (b). The rate constants and the average occupied volume fraction of the system are the same at both the volumes. REs and the LNA predict no change in the steady state of the system as the volume is decreased. Figure 1: Discreteness-induced inversion effect. The species are monomers (species 1, purple), dimers (species 2, orange), and trimers (species 3, green). They are involved in an open trimerization reaction confined to a compartment of volume Ω . Monomers enter the compartment, bind to other monomers to form dimers, and to dimers to form trimers. All molecules leave the compartment at a constant rate. The spheres represent the molecules, whereas the semi-transparent pink surface represents the arbitrarily shaped compartment to which the molecules are confined. The bar graphs reflect the steady-state mean concentrations (denoted for species i ). When the volume decreases below a critical value Ω 12 , the ratio of the steady-state mean concentrations of monomers (species 1) and dimers (species 2) changes from greater than one to less than one. This inversion effect is induced by an increase in the apparent discreteness of the system as the volume is decreased from ( a ) to ( b ). The rate constants and the average occupied volume fraction of the system are the same at both the volumes. REs and the LNA predict no change in the steady state of the system as the volume is decreased. Full size image Theory of the inversion effect We consider a molecular reaction network confined to a well-stirred compartment of volume Ω and involving the interaction of N distinct chemical species via a number of elementary chemical reactions. We furthermore require that the network be monostable. The vector of macroscopic concentrations at any time t , denoted , can be predicted by solving the REs of the network. This prediction ignores molecular discreteness. Time-evolution equations for the approximate mean concentrations when discreteness is taken into account, effective mesoscopic rate equations (EMREs), have recently been derived from the volume expansion of the CME including terms of the order Ω −1/2 , that is, one order higher than terms leading to the LNA [23] (see Methods section for an introduction to EMREs). This derivation is valid for monostable networks. The instantaneous solution of the EMREs is a vector of mean concentrations denoted . By setting the time derivative in the EMREs (equations (9) and (10) in Methods) to zero, one obtains an expression for the difference between the steady-state mean concentration predictions of the EMREs and REs: where , J s is the Jacobian of the REs, and C s is the covariance matrix (the subscript s denotes evaluation at steady state). The vector is the mean–covariance coupling vector whose l th component is: Here 〈 ɛ wz 〉 is short-hand notation for 〈 ɛ w ɛ z 〉, the entry in the w th row and z th column of the covariance matrix of fluctuations (the steady-state solution of the latter is obtained by solving equation (10) in Methods with the time derivative set to zero). We now focus on the physical interpretation of equation (1). Consider the case where the macroscopic steady state of the system is such that . It follows from equation (1) that if δ 1 > δ 2 , there exists a critical compartment volume Ω 12 =( δ 2 − δ 1 )/( φ 2 − φ 1 ) at which the steady-state mean concentrations of the two species become equal, . For volumes smaller than critical, we have . In other words, although accounting for molecular discreteness always leads to some correction to the RE solutions, it is only below a certain critical volume (that is, a certain copy number of molecules) that these corrections lead to qualitative changes in the steady state of a chemical network. We call this novel transition 'discreteness-induced inversion effect', owing to the inversion in the ranking of the steady-state mean concentrations of two species as the volume crosses the critical threshold. This inversion effect is not predicted by the LNA, because it originates from terms of higher order than Ω 0 . For a system of N distinct chemical species, there are at most N ( N −1)/2 different critical volumes, one for each unique pair of species. The general condition for the existence of a critical volume Ω ij for species i and j is: sign( δ i − δj )=sign( φ i − φ j ). REs and the LNA are qualitatively valid in volumes larger than the maximum of all critical volumes, whereas discreteness-induced effects dominate the steady-state behaviour in sub-critical volumes. A necessary (but not sufficient) condition for the inversion effect to occur is that Δ l in equation (2) is non-zero for some l , that is, that there is at least one bimolecular reaction in the reaction network. Quasi-first-order reactions lead to a very small Δ l and are hence unlikely to cause discreteness-induced inversion. A general three-step recipe for predicting the critical volumes of a chemical network is: (i) derive an expression for the vector using the Jacobian of the REs and the mean–covariance coupling vector given in equation (2), both evaluated at steady state; (ii) obtain an explicit expression from the LNA for the steady-state covariance matrix C s in terms of the steady-state RE concentrations by solving equation (10) in the Methods section with the time derivative set to zero; (iii) obtain the final expressions for the critical volumes of the system by substituting the expression for C s into the one previously obtained for , and inserting the latter in The accuracy of the predicted critical volumes depends on the accuracy of the EMRE estimate of the steady-state mean concentrations when discreteness is taken into account, . From equation (1), it is clear that, if δ i is positive, there exists a breakdown volume of the EMREs for which is zero. For volumes smaller than that, becomes negative, which is not physical. A different breakdown volume exists, in principle, for each species. The above prediction of a critical volume can thus only be trusted if it is significantly larger than the maximum of all breakdown volumes. Trimerization in a small compartment We demonstrate and verify our theoretical predictions by exemplarily considering the molecular assembly of trimers from monomers in a small volume [24] . This example is of relevance in various biological contexts, for example, trimerization of receptor proteins and heat-shock factors [27] , [28] , [29] , and also has applications in nanotechnology, including nano-particle clustering and colloidal crystallization. The trimerization reaction scheme is: The above choice of rate constants reduces the dimensionality of the parameter space and simplifies the algebra. Monomers (X 1 ) are input into the compartment in bursts of size m . The monomers form dimers (X 2 ) that can in turn react with other monomers to form trimers (X 3 ). All three species leave the system at a constant rate. The burst-input mechanism models molecules entering the compartment by active transport rather than by diffusion [30] . This is a common mechanism in biological cells [31] , [6] . For example, in the case of receptor trimerization in the plasma membrane, the burst input stems from the vesicular transport of receptor monomers from exocytic compartments. Experimental evidence suggests that the burst size m can be as large as 1,000 (ref. 6 ). Our system is influenced by intrinsic noise from inherent molecular discreteness and by extrinsic noise due to the burst-input process [5] . The parameter m controls the magnitude of extrinsic noise as a larger m implies larger fluctuations in the monomer concentration on input into the compartment. These input fluctuations are not induced by a process inside the compartment. They are caused by the input process, which is external to the compartment and hence a source of extrinsic noise for the reactions inside the compartment. For now, we consider m to be a time-independent constant. Later, we also study the case where m is itself a stochastic quantity, as it is typically in burst phenomena associated with protein production [32] . We start by calculating the critical volumes of this system using the present theoretical framework, and then validate these predictions against exact stochastic simulations [33] . From the Jacobian of the deterministic REs of this system and equation (2), we find: where . The steady-state values of the relevant correlators are obtained by solving the Lyapunov equation (10) with the time derivative set to zero, leading to: with . The elements of the symmetric, positive semi-definite matrix D can be computed from the macroscopic stoichiometry and rate-function matrices S and F (see Methods), leading to: , , and . The vector in equation (4) can then be expressed in terms of the rate constants and the steady-state solution of the REs. We obtain the three critical volumes of the system by substituting the components of into equation (3). In the interest of simplicity, we did not include reverse reactions for the two bimolecular reactions. The inversion effect exists, with or without them, because they are unimolecular; their addition would, however, modify the critical volumes of the system. Simulations confirm the inversion effect We probe the theoretically predicted discreteness effects by exact stochastic simulations. Details of the latter can be found in Methods. We first study the inversion effect for a particular set of parameters to verify its existence. Then, we scan the parameter space using both simulations and the theoretical expressions previously derived to validate the theory's ability to delineate the regions of parameter space, where RE predictions qualitatively fail. Fig. 2 shows the time evolution of the mean concentrations from both ensemble-averaged stochastic simulations (solid lines) and the REs (dashed lines), for three different compartment volumes Ω =10 3 , 12, 3 with identical rate constants k 0 =1/3, k 1 =0.5, and k 2 =1.0 and a fixed burst size m =30. The discreteness of the system, as quantified by the total number of molecules in the compartment n T , becomes more apparent as the volume decreases. The concentrations from the REs and the mean concentrations from the large-volume, large-copy-number ( Ω =1,000, n T =5,195) stochastic simulations are in good agreement ( Fig. 2a ). The two critical volumes of this system, as predicted by our theory (that is, equation (3), together with equations (4,5,6,7)), are Ω 12 =2.79 and Ω 13 =11.83. Indeed, at a compartment volume of Ω =12 ( Fig. 2b ), the stochastic simulations show that the steady-state mean concentrations of species 1 and 3 are roughly equal. For smaller volumes, the steady-state mean concentration of species 3 is larger than that of species 1 ( Fig. 2c ). The simulations thus verify the existence of the predicted discreteness-induced inversion effect. It is noteworthy that the inversion occurs at a copy number of n T =62, which is relatively large considering that stochastic effects are usually deemed significant only in conditions characterized by a mere few molecules. The inversion effect between species 1 and 2, which is theoretically predicted to occur at a smaller volume than that between species 1 and 3, is not found in our simulations ( Fig. 2c ). We will come back to this point later. 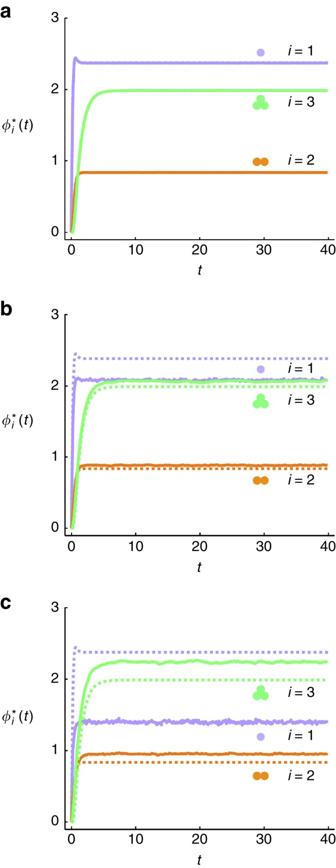Figure 2: Simulations confirming the existence of the inversion effect. Ensemble-averaged mean concentrations versus time for the trimerization reaction confined to three different compartment volumes: (a)Ω=1,000, (b)Ω=12, and (c)Ω=3. The data (solid lines) are obtained from exact stochastic simulations whereas the dashed lines show the RE predictions. Time is in non-dimensional units. The colour coding is purple for monomers, orange for dimers, and green for trimers. The rate constants are fixed tok0=1/3,k1=0.5, andk2=1 and the input burst size tom=30. Given these parameter values, the total number of molecules in the compartment,nT, according to the REs is 5,195 for (a), 62 for (b), and 16 for (c). The simulations confirm the existence of a discreteness-induced inversion below a critical volumeΩ13=11.83 for species 1 and 3. The average concentration of monomers in free and bound states is constant across all volumes,, as is also the occupied volume fraction. This is enforced by steady-state conditions (see Methods). Figure 2: Simulations confirming the existence of the inversion effect. Ensemble-averaged mean concentrations versus time for the trimerization reaction confined to three different compartment volumes: ( a ) Ω =1,000, ( b ) Ω =12, and ( c ) Ω =3. The data (solid lines) are obtained from exact stochastic simulations whereas the dashed lines show the RE predictions. Time is in non-dimensional units. The colour coding is purple for monomers, orange for dimers, and green for trimers. The rate constants are fixed to k 0 =1/3, k 1 =0.5, and k 2 =1 and the input burst size to m =30. Given these parameter values, the total number of molecules in the compartment, n T , according to the REs is 5,195 for ( a ), 62 for ( b ), and 16 for ( c ). The simulations confirm the existence of a discreteness-induced inversion below a critical volume Ω 13 =11.83 for species 1 and 3. The average concentration of monomers in free and bound states is constant across all volumes, , as is also the occupied volume fraction. This is enforced by steady-state conditions (see Methods). Full size image Regions of parameter space where RE models fail To further test the theory, we consider the ( Ω , m )-space where Ω and m take values between 1 and 1,000 in increments of 10. These two parameters are convenient because Ω provides a measure of the intrinsic noise whereas m measures extrinsic noise. The constants k 1 and k 2 are fixed to the same values, as in the previous example. The parameter k 0 is determined by the condition mk 0 / k 2 =10, which guarantees that the comparison between the RE and EMRE is performed at constant volume fraction at all points in parameter space (see Methods). As k 0 m is a constant, the deterministic RE prediction is independent of ( Ω , m ). In contrast, the magnitude of intrinsic and extrinsic noise varies from one ( Ω , m ) to another, leading us to expect inversions in some regions of parameter space, but not in others. Simulations are performed for 100×100 pairs of ( Ω , m ) values. The dark grey and light grey regions in Fig. 3a show where the simulations gave zero and one inversions, respectively. The dashed orange line shows the theoretical prediction of the critical volume Ω 13 as a function of m , calculated using equation (3), together with equations (4,5,6,7). The line accurately demarcates the dark grey and light grey regions, thus validating the theory's ability to predict where the deterministic RE model qualitatively fails. This is also significant from a computational point of view, because the theoretical prediction can be performed much faster than scanning the parameter space in Fig. 3 using a stochastic simulation algorithm (SSA). The dashed red line shows the theoretically predicted critical volume Ω 12 as a function of m , which should demarcate the regions of one and two inversions. However, simulations show that there is no second inversion in the parameter space (a similar observation, but for specific parameters, was pointed out in the previous example of Fig. 2 ). One can see, in Fig. 3a , that the EMRE prediction of a second inversion, as given by the dashed red line, occurs near the white region, where the EMRE predicts negative steady-state mean concentrations. It is hence clear that the inversion is not found by simulations because Ω 12 is too close to the breakdown volume of the EMRE, as previously discussed. 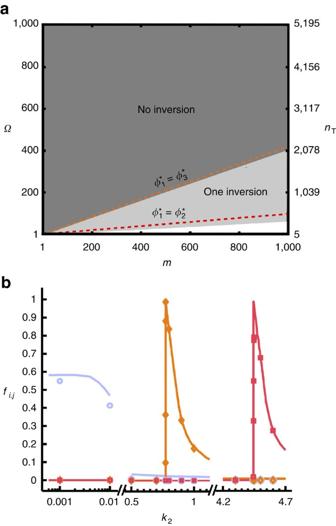Figure 3: Regions of parameter space where REs fail. In (a), we consider the (Ω,m) parameter space. There is a one-to-one correspondence between the volumeΩandnT, the total number of molecules according to the REs. The latter is shown on the right-handyaxis. The dashed lines are the theoretical predictions of the critical volumes. The solid background shading shows the simulation results. Dark grey regions are those where; in this case, there is no inversion, and the RE model is qualitatively correct. Light grey regions are those where; here there exists one inversion, that is, the RE model fails. The demarcation of parameter space by the dashed lines and by the solid shading is almost coincident, highlighting the agreement between theory and simulation. In the white region, the EMRE breaks down as it predicts negative steady-state mean concentrations. This breakdown is induced by very large fluctuations due to the combination of very low copy numbers and large-burst input. (b) Plot of the fractionfi,jof parameter space with at least one inversion between speciesiandjversus the decay rate-constantk2. The peaks identify the conditions of maximal difference between the predictions of deterministic and stochastic models (see text for discussion). In both the panels, the rate constants arek0=10k2/mandk1=0.5, withk2=1 in (a) and varying between 10−3and 4.7 in (b). The colour key is: blue forf1,2, orange forf1,3, and red forf2,3. The data points show the results from exact stochastic simulations33whereas the solid lines show the predictions of the present theory. Figure 3: Regions of parameter space where REs fail. In ( a ), we consider the ( Ω , m ) parameter space. There is a one-to-one correspondence between the volume Ω and n T , the total number of molecules according to the REs. The latter is shown on the right-hand y axis. The dashed lines are the theoretical predictions of the critical volumes. The solid background shading shows the simulation results. Dark grey regions are those where ; in this case, there is no inversion, and the RE model is qualitatively correct. Light grey regions are those where ; here there exists one inversion, that is, the RE model fails. The demarcation of parameter space by the dashed lines and by the solid shading is almost coincident, highlighting the agreement between theory and simulation. In the white region, the EMRE breaks down as it predicts negative steady-state mean concentrations. This breakdown is induced by very large fluctuations due to the combination of very low copy numbers and large-burst input. ( b ) Plot of the fraction f i,j of parameter space with at least one inversion between species i and j versus the decay rate-constant k 2 . The peaks identify the conditions of maximal difference between the predictions of deterministic and stochastic models (see text for discussion). In both the panels, the rate constants are k 0 =10 k 2 / m and k 1 =0.5, with k 2 =1 in ( a ) and varying between 10 −3 and 4.7 in ( b ). The colour key is: blue for f 1,2 , orange for f 1,3 , and red for f 2,3 . The data points show the results from exact stochastic simulations [33] whereas the solid lines show the predictions of the present theory. Full size image The largest critical volume is hence likely to be the only reliable prediction, and also the most important one. This is because the maximum of all critical volumes of a system demarcates the two most important regions: the region where the REs and the LNA correctly predict the ranking of the steady-state mean concentrations, and the region where these predictions are incorrect for at least one pair of species. We also numerically compute maps of the type of Fig. 3a , for other values of the decay constant k 2 . For each value, we compute the fraction f i,j of the ( Ω , m ) space (1 ⩽ ( Ω , m ) ⩽ 1,000) showing inversion of the steady-state mean concentrations of species i and j ( Fig. 3b ). The agreement between EMRE theory (solid lines) and stochastic simulations (data points) is excellent. Consider first the variation of f 1,3 (orange) with k 2 : it is 0 for k 2 ≲ 0.8, and has a sharp peak up to 1 at k 2 ≈0.8, and then decreases smoothly back to zero with further increasing k 2 . The peak value 1 implies that effects due to molecular discreteness can be felt across all of the considered parameter space at that particular value of k 2 . This can be explained as follows: at k 2 =0.77, the macroscopic steady-state concentrations of species 1 and 3 are precisely equal. Discreteness invariably induces a correction to the RE concentrations. Even if this correction is very small, for example, at very large volumes, it is sufficient to break the strict equality between the macroscopic steady-state concentrations of species 1 and 3, and hence to induce an inversion across all of the parameter space. Finite-volume corrections to the macroscopic steady-state concentrations are always non-zero, but they can either amplify or diminish the existing difference between the two macroscopic steady-state concentrations. Of these two cases, the former cannot lead to inversion and occurs for k 2 <0.77, whereas the latter leads to inversion and occurs for k 2 >0.77. This also explains the discontinuous rise of f 1,3 at k 2 =0.77 and the smooth decay beyond this point. The peak in f 2,3 (red) at k 2 =4.45 similarly coincides with the value of k 2 at which the REs predict equal macroscopic steady-state concentrations for species 2 and 3. In contrast, we find no peak in f 1,2 (blue), which monotonically increases as k 2 approaches zero. For the chosen parameter values, the macroscopic steady-state concentration of species 2 monotonically approaches (from below) that of species 1, as k 2 approaches zero. The size of the correction needed to cause inversion hence becomes smaller as k 2 approaches zero. This corresponds to a larger critical volume, which explains the monotonic increase of f 1,2 in the same limit. The general significance of the existence of peaks in f i,j at the point where φ i = φ j is that the region of parameter space where discreteness-induced effects are most conspicuous can be deduced directly from the deterministic REs. Stochasticity in burst size So far, we have assumed that the burst-size parameter m is independent of time. In our model, m could, for example, represent the number of monomers carried by a vesicle in active intracellular transport. Clearly, different vesicles may carry different numbers of monomers, rendering m itself a stochastic variable. We study the effect of stochastic burst sizes using data acquired on burst phenomena in protein production. Experiments have shown that proteins are produced in bursts, where the number of molecules per burst is distributed according to an exponential distribution [32] . We therefore study the situation where the burst size m is sampled, independently for each input event, from a geometric probability distribution, P ( m )= p (1− p ) m −1 , where p =〈 m 〉 −1 , and 〈 m 〉 is the average burst size. This distribution is the discrete analogue of the continuous exponential distribution. We rerun the above parameter scan with stochastic m . The results are shown in Fig. 4 . Comparing Figs 3a and 4 shows that the fraction of parameter space characterized by an inversion is significantly larger when m is a stochastic variable than when m is a time-independent constant. 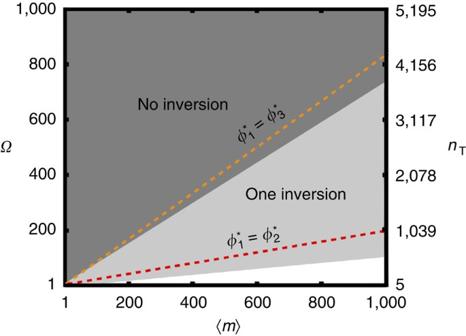Figure 4: Enhancement of inversion effect due to stochasticity in the burst size. We plot the regions of parameter space where the REs fail when the burst sizemis a stochastic variable. The probability distribution of the latter is a geometric distribution with mean 〈m〉. All parameter values and colour codes are the same as inFig. 3a. The dashed lines are the theoretical predictions; the solid background shading shows the simulation results. ComparingFigs 3aand4shows the increase in extrinsic noise caused by makingmstochastic enlarges the portion of parameter space where the REs are qualitatively incorrect (regions of inversion). The theoretical predictions here are obtained using a heuristic modification of the EMRE to approximately account for the randomness in burst size. Figure 4: Enhancement of inversion effect due to stochasticity in the burst size. We plot the regions of parameter space where the REs fail when the burst size m is a stochastic variable. The probability distribution of the latter is a geometric distribution with mean 〈 m 〉. All parameter values and colour codes are the same as in Fig. 3a . The dashed lines are the theoretical predictions; the solid background shading shows the simulation results. Comparing Figs 3a and 4 shows the increase in extrinsic noise caused by making m stochastic enlarges the portion of parameter space where the REs are qualitatively incorrect (regions of inversion). The theoretical predictions here are obtained using a heuristic modification of the EMRE to approximately account for the randomness in burst size. Full size image The new line demarcating the region of no inversion from that characterized by a single concentration inversion can be approximately predicted by a simple, albeit heuristic, modification of the EMREs (see Methods). The two critical volume predictions from the so-modified EMREs are shown as dashed lines in Fig. 4 . The predicted line separating the regions of zero and one inversion (dashed orange line) is in rough agreement with the border between the dark grey and light grey regions obtained from the simulations. The decreased accuracy of the theoretical predictions compared with the case of constant m has two reasons: (i) the present modifications for the EMRE to include stochastic m are heuristic and not derived from first principles; (ii) a stochastic m causes larger fluctuations than a constant m . Terms to order Ω −1/2 , which lead to the EMREs, probably cannot accurately capture the effects of these large fluctuations, presumably requiring higher order terms from the system-size expansion. We have presented and analysed a novel discreteness-induced inversion effect in mesoscopic chemical reaction systems. Our analysis is based on EMREs that only describe monostable chemical reaction networks. This implies that the qualitative change in the steady state at a critical compartment volume is not due to noise-induced transitions between two or more mesoscopic or macroscopic states. Rather, the inversion effect can be explained as follows. According to the CME, the mean rate of a bimolecular reaction between species i and j with concentrations n i Ω −1 and n j Ω −1 , respectively ( n i is number of molecules of species i ), is proportional to the mean of the product of the concentrations, Ω −2 〈 n i n j 〉. Equivalently, it is proportional to the sum of the covariance of concentration fluctuations, , and of the product of the mean concentrations, Ω −2 〈 n i 〉〈 n j 〉. In the limit of large molecule numbers, the covariance becomes very small and the mean rate is simply proportional to the product of the mean concentrations, Ω −2 〈 n i 〉〈 n j 〉; these are the REs. As molecule numbers decrease, the covariance grows and the mean rates of bimolecular reactions deviate from those predicted by the REs, leading to different concentrations. Rates and product concentrations increase if the covariance is positive, and decrease if it is negative. Hence, it is possible that, if the REs predict the steady-state concentration of a species to be larger than that of another species, the reverse may be true for small molecule numbers. This is the presented discreteness-induced inversion effect. Although a few recent papers [34] , [35] , [36] , [37] , [23] , [30] have studied the renormalization of the probability distribution or of the steady-state concentrations with volume, to our knowledge, this is the first time that a discreteness-induced inversion effect has been found and studied in detail. One may ask whether the concentration inversion described here is of importance in any real-world systems. As we show in the Supplementary Methods and Supplementary Discussion , discreteness-induced inversion effects also exist in the protein concentration output of a gene regulation network with negative feedback ( Supplementary Figs S1 and S2 ). This motif is ubiquitous in biology, appearing in such diverse contexts as metabolism [38] , signalling [39] , somitogenesis [40] , and circadian clocks [41] . In biological systems, the gene network considered feeds into more complicated metabolic or signal-transduction networks, and it is plausible that the discreteness-induced concentration inversions at the level of the gene network are propagated into these downstream networks. Practical relevance of the inversion effect requires that the critical volumes be in a physically or physiologically meaningful range. Substituting typical parameter values in equations (3,4,5,6,7): k 0 ∈ [10 2 , 10 4 ]Ms −1 , k 1 ∈ [5×10 4 , 5×10 5 ]M −1 s −1 , k 2 ∈ [10 5 , 10 6 ]s −1 (ref. 42 ), and m =1,000 (ref. 6 ) results in critical volumes in the range 28 nm 3 to 6×10 7 nm 3 (corresponding to spheres of diameters 4 to 500 nm). This suggests that RE predictions may become qualitatively incorrect when modelling chemical reactions inside, for example, lipid rafts (10 to 200 nm (ref. 43 )), endosomes and endocytic vesicles (20 to several hundred nanometers [44] ), sub-organellar structures in the endoplasmic reticulum (few hundred nanometers [45] , [46] ) and mitochondria (few to hundred nanometers, [47] ) and inside 'effective' cytoplasmic compartments (35 to 50 nm (ref. 48 )) created by molecular sieving effects. Similar predictions are expected for reactions occurring in artificial nanoreactors, such as nanofibres, and various biomimetic reactors that typically have diameters of less than a few hundred nanometers [49] , [50] . Effective mesoscopic rate equations Any chemical reaction network proceeding in a well-stirred volume Ω can be written as a set of N distinct chemical species interconverting via R reactions of the type , where j =1,..., R , X i denotes species i ( i =1,..., N ), and s ij and r ij are the stoichiometric coefficients. The j th reaction is characterized by the macroscopic rate constant k j . The constraint Σ i s ij ⩽ 2 ensures that each reaction is at most bimolecular and hence elementary. The deterministic macroscopic REs for this system are of the form: where is the vector of macroscopic concentrations at time t , and ( t ) is the macroscopic rate function. The details of the REs can be encapsulated in two matrices: the N × R stoichiometry matrix S with entries S ij = r ij − s ij and the R × R diagonal matrix F with the j th row equal to . The CME is the corresponding mesoscopic description of the molecular network. Master equations are differential-difference equations [22] whose solution is the probability distribution over the states of the system at time t . The state of the system is the vector of the numbers of molecules of each species (the molecular positions and velocities do not enter the state because of the assumption of well-mixing). Thus, the CME provides a description of chemical processes that accounts for the discrete nature of molecules in well-mixed compartments of mesoscopic to macroscopic sizes. Unfortunately, the stochastic description of a general reaction network given by the CME is not easily amenable to calculation. The problem, however, simplifies if we are only interested in the mean concentrations as predicted by the CME. Approximate time-evolution equations [23] for these mean concentrations have recently been derived from the volume expansion of the CME [1] , including terms up to order Ω −1/2 . Terms of order Ω 0 correspond to the LNA, while terms of order Ω −1/2 and beyond capture the effects of molecular discreteness. These EMREs have the following form for a general reaction network: where we have suppressed the time dependence of variables for clarity. Ω is the volume of the compartment in which the reactions occur, is the vector of mean concentrations (angle brackets denote averaging over an ensemble of independent realizations), and n i is the number of molecules of species i present in the volume Ω . The matrix J is the Jacobian of the REs (equation (8)), and C is the covariance matrix with entries in the i th row and j th column equal to 〈 ɛ i ɛ j 〉, where Ω −1/2 ɛ i is the fluctuation about the macroscopic concentration of species i . The matrix D is given by D = S · F · S T (ref. 13 ) and provides a measure of the strength of the noise. The vector is the mean–covariance coupling vector with components given by equation (2). In the limit of macroscopically large volumes, the Ω −1 term in equation (9) tends to zero, implying that in this limit EMREs reduce to the REs. For mesoscopic volumes, the solution of EMREs is generally different from that of REs. The macroscopic RE prediction for the number of molecules of a species equals the macroscopic concentration of that species multiplied by Ω . It is hence clear that the Ω −1 term in the EMREs arises from the discreteness of the system. Furthermore, inspection of the vector shows that the corrections to the REs are only non-zero if some Jacobian elements in equation (2) are functions of the macroscopic concentrations, that is, if the chemical network has at least one bimolecular reaction. Although EMREs are derived from the CME, they can be constructed from sole knowledge of the REs. The correct way of interpreting the EMREs (equations (9) and (10)) is that given a set of reactions occurring in a volume Ω , is the concentration prediction if we ignore molecular discreteness, and is the approximate mean concentration prediction, if we take discreteness into account. This interpretation comes from the fact that terms of order Ω 0 in the CME's volume expansion do not explicitly depend on Ω , whereas terms of order Ω −1/2 , from which the EMREs are obtained, do depend on Ω (see equation 14 in ref. 23 ). Considering terms of even higher order in the volume expansion may reveal further discreteness-induced effects that cannot be captured by EMREs. The EMREs can also be heuristically modified to describe scenarios with stochasticity in the burst size parameter, such as that studied in the preceding sections. In this case, the REs are also stochastic and their average solutions must be obtained by ensemble-averaging over a large number of independent realizations. The concentrations φ 1 and φ 2 to be used in the EMREs (equations (6,7,8,9,10)) are then set to the averaged concentrations from the stochastic REs. Furthermore, the EMREs explicitly depend on m via D 11 . We hence replace m 2 in D 11 with its average computed over the geometric distribution, that is, 〈 m 2 〉=〈 m 〉(2〈 m 〉−1). Simulation details The theoretical predictions of the critical volumes, at which the trimerization system undergoes inversion, are validated using the partial-propensity direct method [33] , an exact SSA that produces sample trajectories from the CME at a fraction of the computational cost incurred by traditional SSA formulations. The volume dependence enters the stochastic simulation through the propensity functions of the input and bimolecular reactions, which scale as Ω and 1/ Ω , respectively, in accordance with the CME [1] . We compute steady-state mean concentrations from the simulations by ensemble-averaging the number of molecules of species i over 2×10 4 independent realizations, and dividing by Ω . Steady-state conditions require that for all volumes the influx of monomers equals their efflux, that is, . The efflux is equal to the sum of three terms: the first is the efflux of monomers, the second is the efflux of monomers that are part of a dimer, and the third is the efflux of monomers that are part of a trimer. This condition is also valid for the deterministic REs, that is, mk 0 = k 2 ( φ 1 +2 φ 2 +3 φ 3 ). Hence, the total steady-state mean concentration of monomers (in free form or bound in dimers and trimers), , is equal to mk 0 / k 2 , where N m is the total number of monomers, that is, . We study independent realizations of the same chemical reaction system in compartments of different volumes. This implies that mk 0 / k 2 is a volume-independent constant and that there exists a linear relationship between N m and Ω. One can also show that the constant mk 0 / k 2 is equal to Φ / v , where v is the physical volume of a single monomer and Φ is the average occupied volume fraction at steady state. Realizations in different volumes have equal occupied volume fractions, and the relationship between N m and Ω can be written as Ω =( v /Φ) N m . The quantity N m is only an upper bound on the actual number of discrete molecules in the system. Hence, instead of using N m as a measure of system discreteness, we use the total number of molecules as predicted by the REs: n T =Ω( φ 1 + φ 2 + φ 3 ). A smaller n T indicates higher discreteness, and vice versa . How to cite this article: Ramaswamy, R. et al . Discreteness-induced concentration inversion in mesoscopic chemical systems. Nat. Commun. 3:779 doi: 10.1038/ncomms1775 (2012).